High-quality monolayer superconductor NbSe2grown by chemical vapour deposition The discovery of monolayer superconductors bears consequences for both fundamental physics and device applications. Currently, the growth of superconducting monolayers can only occur under ultrahigh vacuum and on specific lattice-matched or dangling bond-free substrates, to minimize environment- and substrate-induced disorders/defects. Such severe growth requirements limit the exploration of novel two-dimensional superconductivity and related nanodevices. Here we demonstrate the experimental realization of superconductivity in a chemical vapour deposition grown monolayer material—NbSe 2 . Atomic-resolution scanning transmission electron microscope imaging reveals the atomic structure of the intrinsic point defects and grain boundaries in monolayer NbSe 2 , and confirms the low defect concentration in our high-quality film, which is the key to two-dimensional superconductivity. By using monolayer chemical vapour deposited graphene as a protective capping layer, thickness-dependent superconducting properties are observed in as-grown NbSe 2 with a transition temperature increasing from 1.0 K in monolayer to 4.56 K in 10-layer. Monolayer superconductors provide ideal models for investigating superconductivity in the two-dimensional (2D) limit, as well as superconductor-substrate interplay [1] , [2] , [3] , [4] , [5] . Strong enhancement of the transition temperature ( T c ) has been reported in the monolayer FeSe/SrTiO 3 system [6] , [7] , which indicates that 2D ultra-thin films have the potential to be high- T c superconductors. However, the superconductivity in most monolayers (Pb [8] , [9] , In [8] , [10] , FeSe [6] ) only survives on certain substrates, probably due to particular interface bonds [6] , [8] . Monolayer NbSe 2 , has recently been recognized as an intrinsic monolayer superconductor, due to the occurrence of superconductivity without the need of a special substrate [4] . NbSe 2 crystallizes in the same layered hexagonal structure as 2 H -MoS 2 , where the niobium atoms sit at the center of trigonal selenium prisms. Compared with the bulk, 2D NbSe 2 exhibits significantly different properties arising from reduced dimensionality, as exemplified by the observation of Ising superconductivity [11] , quantum metallic state [12] , and strong enhancement of charge density wave order [4] . Defects in an ultrathin superconductor are known to be a critically detrimental factor to intrinsic 2D superconductivity [13] , [14] . Monolayer ambient-sensitive [15] , [16] NbSe 2 is predisposed to receive defects from the substrate and ambient environment. Therefore, the growth of superconducting NbSe 2 monolayers is a great challenge. Though superconducting NbSe 2 layers can be mechanically exfoliated from bulk NbSe 2 crystals, it is not a scalable method. Also, the thickness and size of exfoliated NbSe 2 flakes cannot be controlled. In the past few years, chemical vapour deposition (CVD) has been widely employed to synthesize ultrathin semiconducting transition metal dichalcogenides (TMDs) such as MoS 2 and WSe 2 [17] , [18] , [19] , [20] , [21] , [22] , [23] , [24] . Recently, NbSe 2 multilayers were prepared by selenizing pre-deposited Nb 2 O 5 films. However, none of the prepared NbSe 2 was found to be superconducting [25] , [26] , probably due to the large concentration of defects created during growth. Currently, superconducting NbSe 2 monolayers can only be grown by molecular beam epitaxial (MBE) under ultrahigh vacuum (UHV) and on a dangling bond-free graphene or h -BN substrate [3] , [27] , in order to minimize environment- and substrate-induced disorders/defects. However, MBE is expensive to perform because it requires a high-priced apparatus and a UHV environment. Furthermore, MBE growth of NbSe 2 is only available on specific graphene and h -BN substrates [3] , [27] , and the individual domain size is < 1 µm [3] , [27] . Therefore, it is desirable to develop a facile growth method to produce high-quality superconducting NbSe 2 layers. In this work, we report the growth of the monolayer superconductor NbSe 2 at ambient pressure on a variety of substrates. Atomic-resolution annual dark-field scanning transmission electron microscope (ADF-STEM) imaging reveals the atomic structure of the intrinsic defects in the as-grown monolayer NbSe 2 crystal, such as point defects and grain boundaries, and confirms the low concentration of defects in both mono- and few-layer regions. Transport data indicate that even low concentration of defects exist in CVD-grown NbSe 2 , they will not significantly affect the superconducting properties. Growth of monolayer NbSe 2 crystals Atomically thin NbSe 2 crystals were grown on diverse substrates by ambient pressure CVD in a tube furnace (Supplementary Fig. 1 ). Partially oxidized niobium powder NbO x ( x ≤ 2.5) was chosen as the precursor (Supplementary Fig. 2 ). Briefly, the powder mixture of NbO x and NaCl was loaded in an alumina boat into the center of a fused quartz tube. Diverse substrates (SiO 2 /Si, Si(100), quartz, etc.) were placed 1-3 mm above the powder mixture with the polished side faced down. Selenium powder was located at the entrance of the tube furnace, where the temperature was 300–340 °C during growth. Further details of the experiments are provided in the “Methods” section. 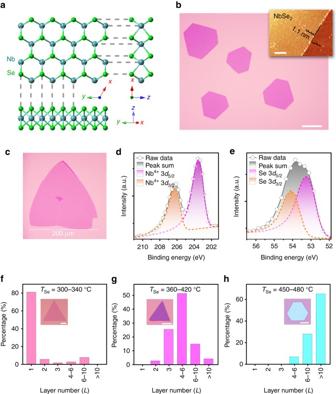Fig. 1 Atomic structure, morphologies, and characterizations of NbSe2crystals.aBall-and-stick model of monolayer 2H-NbSe2viewed from three different directions.bOptical image of uniform NbSe2crystals deposited on a SiO2/Si substrate.Scale bar, 40 µm. A representative AFM image (inset;scale bar, 1 µm) shows the typical thickness is 1.1 nm.cA monolayer NbSe2crystal with edge length of 0.2 mm.d,eX-ray photoemission spectroscopy (XPS) spectra of thedNb 3dandeSe 3dpeaks from NbSe2crystals deposited on SiO2/Si substrate.f–hStatistic thickness distributions and representative morphologies (inset) of NbSe2crystals synthesized withTSesetting atf300-340,g360-420 andh450-480 °C, respectively.Scale barsfrominsetoff–hare 20, 5 and 5 µm. Thickness ofinsetcrystals off–hare 1.1, 5.1 and 16.2 nm Figure 1a shows the crystal structure of monolayer NbSe 2 viewed from different angles. The as-deposited NbSe 2 crystals on SiO 2 /Si are typically triangular or hexagonal in shape. Figure 1b shows the optical image of uniform hexagonal NbSe 2 crystals. A representative atomic force microscopy (AFM) measurement ( inset of Fig. 1b ) indicates the thickness of the NbSe 2 crystal is around 1.1 nm, which corresponds to a monolayer TMD [20] , [28] . As shown in Fig. 1c , the lateral domain size of monolayer CVD-grown NbSe 2 can reach 0.2 mm, which is ~10 2 times as large as that of NbSe 2 prepared by MBE (<1 µm) [3] , [27] . In addition to SiO 2 /Si substrates, our CVD method can deposit NbSe 2 layers on arbitrary selenium-resistant crystalline and amorphous substrates, such as silicon (100), quartz, and CVD graphene (Supplementary Fig. 3 ). Different substrates may result in NbSe 2 flakes of varied morphologies (Supplementary Figs. 3 and 4 ), suggesting that the underlying substrate has an influence on the nucleation and growth of NbSe 2 . Direct growth on diverse substrates makes it feasible to study the NbSe 2 -substrate interaction and related properties. Fig. 1 Atomic structure, morphologies, and characterizations of NbSe 2 crystals. a Ball-and-stick model of monolayer 2 H -NbSe 2 viewed from three different directions. b Optical image of uniform NbSe 2 crystals deposited on a SiO 2 /Si substrate. Scale bar , 40 µm. A representative AFM image ( inset ; scale bar , 1 µm) shows the typical thickness is 1.1 nm. c A monolayer NbSe 2 crystal with edge length of 0.2 mm. d , e X-ray photoemission spectroscopy ( XPS ) spectra of the d Nb 3 d and e Se 3 d peaks from NbSe 2 crystals deposited on SiO 2 /Si substrate. f – h Statistic thickness distributions and representative morphologies ( inset ) of NbSe 2 crystals synthesized with T Se setting at f 300-340, g 360-420 and h 450-480 °C, respectively. Scale bars from inset of f – h are 20, 5 and 5 µm. Thickness of inset crystals of f – h are 1.1, 5.1 and 16.2 nm Full size image The chemical states of the as-grown NbSe 2 samples were examined by X-ray photoemission spectroscopy (XPS) (Supplementary Fig. 5 ). Figure 1d is the Nb 3 d core-level spectrum, and the two peaks at 203.4 and 206.1 eV can be assigned to Nb 4+ 3 d 5/2 and Nb 4+ 3 d 3/2 of NbSe 2 [29] . The absence of Nb 5+ 3 d 5/2 and Nb 5+ 3 d 3/2 peaks at higher binding energy (from 207.3 to 211.0 eV) indicates that the sample was not oxidized [30] . The Se 3 d core levels spectrum can be fitted with Se 3 d 5/2 (53.2 eV) and Se 3 d 3/2 (54.1 eV) peaks in agreement with the spectra of NbSe 2 (Fig. 1e ) [29] , [30] . Furthermore, the absence of Na 1 s and Cl 2 p peaks suggests that as-grown NbSe 2 was not contaminated by the NaCl precursor (Supplementary Fig. 6 ). Tuning the thickness of NbSe 2 layers In addition to producing monolayer NbSe 2 , the proposed CVD method is also capable of acquiring NbSe 2 crystals with different thicknesses from 1.1 to 16 nm, which will be useful for investigating the thickness-dependent properties such as superconductivity, charge–density-wave order and their interplay in the 2D system. The NbSe 2 layer thickness was found to be sensitive to the heating temperature of selenium source ( T Se ). A portable thermocouple thermometer was used to measure the selenium temperature during sample growth. Figure 1f-h shows the thickness distribution statistics and representative morphologies ( inset of Fig. 1f-h and Supplementary Fig. 7 ) of NbSe 2 crystals grown with T Se of (f) 300–340, (g) 360–420, and (h) 450–480 °C, respectively, while keeping all other growth parameters identical. Notably, the average thickness of obtained NbSe 2 increased with T Se . Monolayer NbSe 2 crystals were obtained only when selenium was heated to 300–340 °C. In our experimental set-up, relatively higher T Se will induce a higher flow rate of the selenium vapour. Therefore, these results indicate that the thickness of NbSe 2 films highly relies on the flow rate of the selenium vapour. Supplementary Fig. 8 shows AFM images of NbSe 2 crystals with different thicknesses up to 16.2 nm. Raman spectra of the as-grown crystals show two characteristic peaks of NbSe 2 (Supplementary Fig. 9 ), including the in-plane E 2g mode at about 250 cm −1 and the out-of-plane A 1g mode at about 225 cm −1 . The broad feature at about 180 cm −1 is described as a soft mode because of its frequency behavior with temperature [4] , [31] . Thickness dependence of the Raman spectra of NbSe 2 is also shown in Supplementary Fig. 9 . For monolayer NbSe 2 , the Raman intensity of both A 1g and E 2g are very weak at room temperature. With the sample thickness increases, the intensity of A 1g and E 2g increase significantly. Structural characterization In order to examine the quality of the as-grown 2 H -NbSe 2 atomic layers, the atomic structure and the chemical composition of the NbSe 2 layers were characterized by atomic resolution ADF-STEM imaging, electron energy-loss spectroscopy (EELS) and energy-dispersive X-ray spectrometry (EDX). Since a bare NbSe 2 monolayer film is sensitive to the ambient environment, we transferred the NbSe 2 flakes grown on SiO 2 substrate with graphene encapsulation (see “Methods” section), constructing a graphene/NbSe 2 /graphene sandwich structure for STEM imaging. Such structures have been demonstrated to be effective in protecting sensitive monolayer materials from being oxidized [32] . 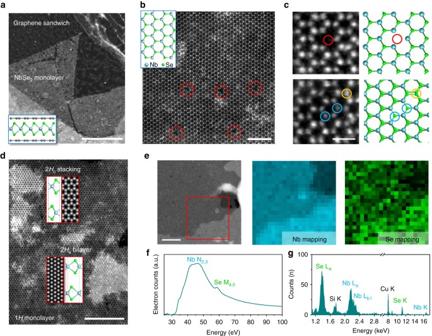Fig. 2 ADF-STEM images, EELS, and EDX characterizations of the as-synthesized NbSe2atomic layers.aA low magnified annular dark-field scanning transmission electron microscope (ADF-STEM) image showing a large region of monolayer NbSe2encapsulated by the graphene sandwich. The schematic is shown in theinset.bAtomic resolution ADF-STEM image of the hexagonal NbSe2lattice. Diselenium vacancies are highlighted byred circles. Theinsetof panelbshows the structural model of 2H-NbSe2, withcyanandgreen colorindicating Nb and Se atoms, respectively.cDifferent point defects in monolayer NbSe2and their atomic models. Diselenium vacancy, monoselenium vacancy, and anti-site defect SeNbare highlighted byred,blue, andyellow circles, respectively.dAtomic resolution ADF-STEM image of two bilayer islands in NbSe2, showing the coexistence of 2Haand 2Hcstacking sequence. Theinsetsare corresponding atomic models and simulated STEM images.eSTEM image of a large region of NbSe2used for the collection of electron energy-loss spectroscopy (EELS) and energy-dispersive X-ray spectrometry (EDX) spectra. The collected region is highlighted inred square. Nb and Se EELS mapping are provided next to it.fTypical EELS andgEDX spectra of the region shown ine. The Cu signal in the EDX spectra comes from the Cu grid.Scale bars, 500 nm (a), 2 nm (b), 0.5 nm (c), 5 nm (d), 50 nm (e) Figure 2a shows a low magnification ADF-STEM image of a large area of monolayer NbSe 2 sandwiched by graphene (schematic shown in the inset ), where little oxidization is observed. Figure 2b shows a zoom-in image of the same area with atomic resolution, displaying the hexagonal atomic lattice of alternating bright and dark spots, which corresponds, respectively, to the Se 2 and Nb atomic columns as indicated in the atomic model, confirming its hexagonal phase. Diselenium vacancy can be directly visualized by their distinguishable contrast within the image, as highlighted by the red circles . Since the STEM image contrast is directly related to the atomic number and the number of atoms of the imaged species, more types of intrinsic point defects can be identified by carefully examining the image contrast of each atomic column. Figure 2c shows the atomic resolution image of three major types of point defects found in the monolayer NbSe 2 film, which are diselenium vacancy ( \({{\rm{V}}_{{\rm{S}}{{\rm{e}}_{\rm{2}}}}}\) , red ), monoselenium vacancy (V Se , blue ), and anti-site defect where a Se 2 column replaces the Nb ( yellow ). These intrinsic point defects are similar to those found in MoS 2 and MoSe 2 with the same hexagonal phase [33] , [34] grown by CVD method. We can therefore calculate the defect concentration in certain area by counting the number of point defects. The defect concentration in Fig. 2b is estimated to be ~0.18 nm −2 , which is similar to the case in mechanical exfoliated monolayer materials [35] , demonstrating the sufficiently low defect concentration in the film grown by our CVD method. The defect concentration is similar in multiple layer of NbSe 2 , as shown in Supplementary Fig. 10 . Fig. 2 ADF-STEM images, EELS, and EDX characterizations of the as-synthesized NbSe 2 atomic layers. a A low magnified annular dark-field scanning transmission electron microscope ( ADF-STEM ) image showing a large region of monolayer NbSe 2 encapsulated by the graphene sandwich. The schematic is shown in the inset . b Atomic resolution ADF-STEM image of the hexagonal NbSe 2 lattice. Diselenium vacancies are highlighted by red circles . The inset of panel b shows the structural model of 2 H -NbSe 2 , with cyan and green color indicating Nb and Se atoms, respectively. c Different point defects in monolayer NbSe 2 and their atomic models. Diselenium vacancy, monoselenium vacancy, and anti-site defect Se Nb are highlighted by red , blue , and yellow circles , respectively. d Atomic resolution ADF-STEM image of two bilayer islands in NbSe 2 , showing the coexistence of 2 H a and 2 H c stacking sequence. The insets are corresponding atomic models and simulated STEM images. e STEM image of a large region of NbSe 2 used for the collection of electron energy-loss spectroscopy ( EELS ) and energy-dispersive X-ray spectrometry ( EDX ) spectra. The collected region is highlighted in red square . Nb and Se EELS mapping are provided next to it. f Typical EELS and g EDX spectra of the region shown in e . The Cu signal in the EDX spectra comes from the Cu grid. Scale bars , 500 nm ( a ), 2 nm ( b ), 0.5 nm ( c ), 5 nm ( d ), 50 nm ( e ) Full size image We further study the stacking sequence in the CVD-grown NbSe 2 sample. Figure 2d shows two stacking orders that coexist in the bilayer region. While the lower bilayer is confirmed to be in 2 H a stacking, which is a stacking type commonly found in bulk NbSe 2 , where Nb atoms are aligned to each other between the layers (atomic model in the inset ), the upper bilayer is revealed to be in 2 H c stacking, similar to the 2 H stacking in MoS 2 . This is further evidenced by the equal intensity of each atomic column in the hexagonal rings, suggesting all the Nb atoms are aligned with the Se 2 columns between the layers. Nevertheless, we found the dominating stacking in bilayers is the 2 H a stacking phase. This result implies that, though 2 H c stacking is rarely seen in bulk, it can still form in the CVD process presumably due to the weak van der Waal interlayer interaction, which can be overcome by the rapid nucleation process. EDX and EELS were used to identify the chemical constituents of the as-grown layers. Figure 2e shows the region that is used to perform the EDX and EELS experiment. Both EDX and EELS unambiguously show the as-grown NbSe 2 film only contains Nb and Se without the presence of any other impurities (Fig. 2f, g ). Similar defect and stacking structures are also observed in the NbSe 2 layers that are directly grown on graphene substrate, as shown in Supplementary Fig. 11 . Due to the protection of the graphene sandwich structure, we were able to directly observe the grain boundary structure in the air-sensitive NbSe 2 monolayer grown on SiO 2 /Si by CVD method. 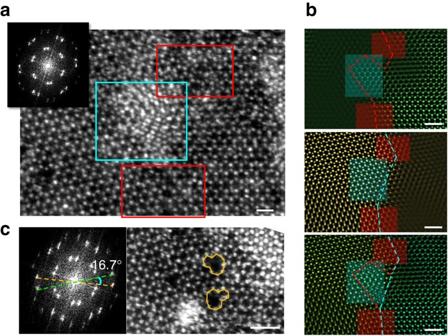Fig. 3 ADF-STEM images of the grain boundary in monolayer NbSe2.aA tilted grain boundary with misorientation angle of 11°. Both atomically sharp lateral interconnected (red rectangle) and vertically stacked (blue rectangle) boundary regions are found to coexist. Theinsetshows the fast Fourier transformation (FFT) of the image. The distorted polygons are also highlighted in thered rectangle.Scale bar, 0.5 nm.bSelected FFT-filtered image of the two domains and their overlap images. The overlapped image confirms the coexistence of the two types of grain boundaries.Scale bar, 1 nm.cSimilar tilted grain boundary without an overlapping region nearby. Theorange linesindicate the five-seven dislocation pairs, which is consistent with the theoretical predictions of the grain boundary structure.Scale bar, 1 nm Figure 3a displays a tilted grain boundary with a small misorientation angle (about 11°, determined by fast Fourier transform (FFT) in the inset ). Interestingly, we found that two types of grain boundary structures coexist, as highlighted by different colored rectangles. The red region indicates the boundary that is atomically sharp, where two domains connects by distorted polygons to accommodate the strain due to the misorientation. The blue region represents another type of boundary, where the two domains overlap with each other, forming a vertically stacked structure. This is further evidenced by the selected FFT-filtered image shown in Fig. 3b , in which the two domains are separated according to the misorientation angles. Although both types of boundaries have been reported previously [36] , [37] , [38] , it is commonly believed that only one of them can be formed depending on the dynamic energy between the growing frontiers of the misoriented domains during the growth process. The coexistence of both types in a single grain boundary structure suggests the formation energy between these two types of structures (atomically sharp and vertically stacked) is similar in NbSe 2 , where their co-growth can be induced by local fluctuation of the growing conditions. Figure 3c shows a similar tilted grain boundary without overlapping regions nearby. The ideal five-seven dislocation pairs are found periodically embedded along the grain boundary (highlighted by orange outline ), which is similar to the case of other TMD materials [34] , [37] and consistent with the theoretical predictions [39] . In contrast, the polygons are found to be more distorted and did not have a periodic distribution when the overlapping boundary is nearby, as shown in the red rectangular regions in Fig. 3a . This may be due to the alternation of the local strain profile in the atomically sharp grain boundary region induced by the overlapping area, which leads to the random formation of distorted polygons to release the inhomogeneous strain. These results reveal the local atomic structure of the grain boundaries, for the first time, in air-sensitive monolayer NbSe 2 which is hard to observe due to its easy oxidization without any protection. Fig. 3 ADF-STEM images of the grain boundary in monolayer NbSe 2 . a A tilted grain boundary with misorientation angle of 11°. Both atomically sharp lateral interconnected ( red rectangle ) and vertically stacked ( blue rectangle ) boundary regions are found to coexist. The inset shows the fast Fourier transformation ( FFT ) of the image. The distorted polygons are also highlighted in the red rectangle . Scale bar , 0.5 nm. b Selected FFT-filtered image of the two domains and their overlap images. The overlapped image confirms the coexistence of the two types of grain boundaries. Scale bar , 1 nm. c Similar tilted grain boundary without an overlapping region nearby. The orange lines indicate the five-seven dislocation pairs, which is consistent with the theoretical predictions of the grain boundary structure. Scale bar , 1 nm Full size image Transport properties of mono- and few-layer NbSe 2 To further characterize the quality and dimensionality of as-grown NbSe 2 crystals, a low-temperature transport experiment was carried out on Hall-bar devices. Because of its air sensitivity [15] , ultrathin NbSe 2 was first covered with a continuous monolayer graphene film before device fabrication (see “Methods” section). 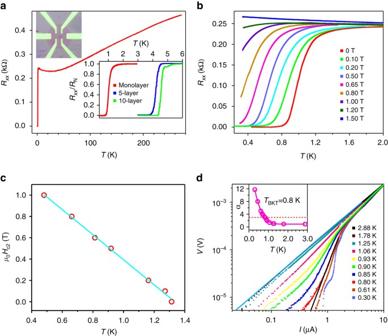Fig. 4 Superconductivity in monolayer NbSe2devices.aTemperature dependence of the longitudinal resistanceRxxfor sample A—a monolayer NbSe2device.Upper left inset: Optical image of a typical graphene protected monolayer NbSe2device.Lower right inset: Superconductivity in monolayer, 5-layer and 10-layer NbSe2devices.bSuperconductivity of sample A in different magnetic fields.cTemperature dependence of the upper critical fieldHc2. Thesolid lineis the linear fit toHc2.dVoltage–current (V-I) characteristic at different temperatures on a logarithmic scale. Thesolid blue lineindicates the Ohmic behavior at high temperature. Thesolid black linerepresents the expectedV∝I3behavior at the Berezinskii-Kosterlitz-Thouless (BKT) transition. Theinsetshows the temperature-dependent exponent deduced from the power-law behavior,V∝Iα. As indicated by thered dashed line,αapproaches 3 atT =0.8 K 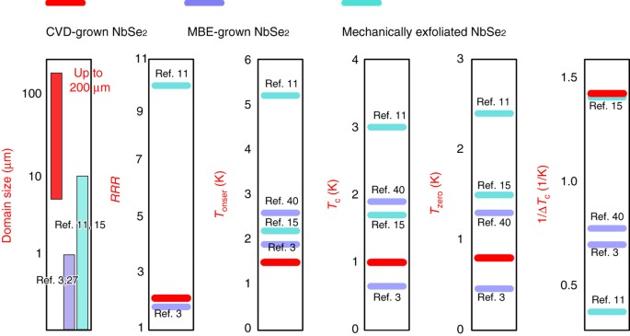Fig. 5 Comparison of the superconducting performance of monolayer NbSe2prepared by CVD and other methods. Fromlefttoright: domain size, residual resistance ratio RRR,Tonset,Tc(0.5 RN),Tzero, and1/ΔTcfor monolayer NbSe2samples prepared with different methods Figure 4a shows the temperature T dependence of longitudinal resistance R xx for sample A—a representative monolayer NbSe 2 device (see Supplementary Note 1 and Supplementary Fig. 12 for more devices and data) at zero magnetic field. Consistent with previous studies [3] , [11] , [12] , the sample shows a metallic behavior (d R /d T > 0) at high temperatures. At T onset = 1.5 K, R xx begins to decrease sharply and drops to zero at T zero = 0.8 K, indicating the occurrence of superconductivity. Additionally, we find the superconducting transition in our high-quality NbSe 2 crystals can be tuned by changing the sample thickness. The lower right inset of Fig. 4a displays the normalized resistance R xx / R N as a function of temperature for NbSe 2 with different thickness. It is evident that the superconducting transition critical temperature T c (0.5 R N ) can be tuned from 4.56 K for 10-layer, 4.2 K for 5-layer, to 1.0 K for monolayer. Due to its sensitivity to moisture and oxygen, even when protected by graphene, the superconductivity of NbSe 2 sample degrades with increasing ambient exposure (Supplementary Fig. 13 and Supplementary Table 1 ), which is discussed in Supplementary Note 2 . Fig. 4 Superconductivity in monolayer NbSe 2 devices. a Temperature dependence of the longitudinal resistance R xx for sample A—a monolayer NbSe 2 device. Upper left inset : Optical image of a typical graphene protected monolayer NbSe 2 device. Lower right inset : Superconductivity in monolayer, 5-layer and 10-layer NbSe 2 devices. b Superconductivity of sample A in different magnetic fields. c Temperature dependence of the upper critical field H c2 . The solid line is the linear fit to H c2 . d Voltage–current ( V - I ) characteristic at different temperatures on a logarithmic scale. The solid blue line indicates the Ohmic behavior at high temperature. The solid black line represents the expected V ∝ I 3 behavior at the Berezinskii-Kosterlitz-Thouless (BKT) transition. The inset shows the temperature-dependent exponent deduced from the power-law behavior, V ∝ I α . As indicated by the red dashed line , α approaches 3 at T = 0.8 K Full size image To compare the quality of the monolayer NbSe 2 prepared with different methods, the residual resistance ratio (defined as the ratio of the room temperature resistance R 300 K to the normal-state resistance R N ) RRR, the superconducting transition onset temperature T onset , the critical temperature T c (0.5R N ), the zero-resistance temperature T zero , and the inverse of the superconducting transition width 1/ Δ T c are summarized in Fig. 5 . It is noted that our CVD-grown monolayer NbSe 2 has a RRR = 2.0 very close to the reported value for MBE-grown NbSe 2 [3] , but the CVD sample has a T zero (0.8 K) almost two times as high as that of MBE NbSe 2 [3] . Though a much higher zero-resistance temperature T zero = 1.3 K was reported in Se-capped MBE-grown monolayer NbSe 2 , however, the resistance did not really drop to zero [40] . Besides, the Δ T c in the CVD-grown sample is only 0.7 K, which is superior to all reported MBE NbSe 2 [3] , [40] and comparable to the best record in mechanically exfoliated samples [15] . The above data indicate that the CVD-grown NbSe 2 samples are high quality. Fig. 5 Comparison of the superconducting performance of monolayer NbSe 2 prepared by CVD and other methods. From left to right : domain size, residual resistance ratio RRR, T onset , T c (0.5 R N ), T zero , and 1/ Δ T c for monolayer NbSe 2 samples prepared with different methods Full size image Figure 4b shows the temperature and field dependence of R xx for sample A (see Supplementary Note 1 for more devices and data) with the field perpendicular to the sample plane. Under a magnetic field, the critical temperature T c is defined by where the resistance is 90% of the normal state value R N . With increasing the strength of magnetic field B , T c shifts to lower temperatures. Finally, the superconductivity is completely suppressed with a magnetic field of about 1.5 T at T = 0.3 K. We summarize the H c2 - T c phase diagram, where H c2 is the upper critical field, in Fig. 4c and find a linear relationship between H c2 and T c , which is a characteristics of 2D superconductors [11] , [12] , [13] and can be explained by the standard linearized Ginzburg-Landau (GL) theory [41] , \({H_{{\rm{c}}2}}(T) = \frac{{{\phi _0}}}{{2\pi {\xi _{{\rm{GL}}}}{{(0)}^2}}}\left( {1 - \frac{T}{{{T_{\rm{c}}}}}} \right)\) , where \({\xi _{{\rm{GL}}}}\) (0) is the zero-temperature GL in-plane coherence length and \({\phi _0}\) is the magnetic flux quantum. As shown in Fig. 4c , a linear fit between H c2 and T c yields \({\xi _{{\rm{GL}}}}\) (0) = 18 nm (see Supplementary Note 3 and Supplementary Fig. 14 for more transport data of NbSe 2 grown on graphene substrate), which is about twice of the bulk value [16] . Based on the normal state resistance R N and carrier density n s as determined by Hall measurement (Supplementary Note 4 and Supplementary Fig. 15 ), the mean free path l m = 1.3 nm can be obtained, smaller than that in exfoliated sample [12] . On the other hand, the normal state sheet resistance R s = 727 Ω (taken at T onset = 1.5 K) is much smaller than the quantum resistance R q = h /4 e 2 ≈ 6.45 kΩ, where e is the electron charge and h is Planck’s constant, above which a disorder-induced superconductor-insulator transition emerges [42] . The above discussions indicate that our sample is in the low-disorder regime [11] , [13] , [40] . For a 2D superconductor with the thickness d < \({\xi _{{\rm{GL}}}}\) (0), the superconducting phase transition is expected to be of the Berezinskii-Kosterlitz-Thouless (BKT) type [43] , [44] . Figure 4d shows voltage–current ( V - I ) behavior as a function of temperature on a log-log scale. The V - I relations change from a linear to a power-law dependence, V ∝ I α at T c (0.5 R N ), which is consistent with expectations for a 2D superconductor based on the theoretical model of the BKT transition. In the inset of Fig. 4d , we plot the exponent α vs. T , which is extracted from the slope of V - I traces. The BKT transition temperature T BKT is estimated to be 0.8 K from where α = 3 interpolates. The above data confirm that monolayer NbSe 2 exhibits the characteristics of a true 2D superconductor. The developed CVD growth technology has enabled the realization of superconductivity in non-UHV grown monolayer materials. Our results also provide a comprehensive understanding of the defect structure, superconducting performance as well as the influence of ambient-induced defects on superconductivity of NbSe 2 . It is evident that even though low concentrations of selenium vacancy-related defects remained in the CVD-grown NbSe 2 , they will not significantly affect the superconducting properties. Our facile CVD technology not only provides an excellent platform for the investigation of many fascinating properties of NbSe 2 , but also holds promise for large-scale synthesis of 2D superconducting NbSe 2 films for potential device applications. Future developments may also include investigation and understanding of NbSe 2 -substrate interplay and related novel properties, inspired by the research on 2D high- T c Fe-chalcogenide superconductors [6] , [7] , [45] (more discussion in Supplementary Note 5 ). More recently, monolayer NbSe 2 was suggested as a candidate for realizing topological superconducting phase and engineering Majorana fermions [46] , [47] . Therefore, the present work offers possibilities for the study of topological physics. More importantly, our work indicates that a UHV environment is not necessarily required for the growth of monolayer superconductors. In our salt-assisted CVD synthesis of NbSe 2 , the role of salt is particularly important as no nucleation of NbSe 2 can be observed without salt. It is noted that all niobium oxides have melting points above 1510 °C, which make them difficult to vaporize and react with selenium in the CVD process. The products of reactions between molten salts and metal (Mo [48] , W [28] , and Nb [49] ) oxides have been investigated by several groups and found to be metal oxychlorides, which have much lower melting points compared with corresponding metal oxides [28] , [48] , [49] . Thus, it is suggested that in our CVD process, NaCl reacts with niobium oxides to give volatile niobium oxychloride [28] , therefore increasing the vapour pressure of precursor and facilitating the growth of NbSe 2 . With the proposed salt-assisted CVD method, a number of other 2D and even monolayer superconductors (2 H -TaS 2 , 2 H -TaSe 2 , 1 T -TiSe 2 , and 1 T -Cu x TiSe 2 , etc.) could be synthesized by substituting niobium oxides with corresponding metal oxides precursors. Considering that most of the mentioned monolayers have never been synthesized (even by MBE) and investigated, the new growth technology will enrich the research field of 2D TMDs superconductivity greatly. Atomically thin NbSe 2 crystals synthesis We used partially oxidized niobium powder NbO x ( x ≤ 2.5) as precursor for growing NbSe 2 . In the first step, 5 g niobium powder (99.8%, 325 mesh, Alfa Aesar) was loaded into a both-ends-opened quartz tube equipped in a tube furnace. The niobium powder was ignited when furnace was heating to about 680 °C. After 1 min combustion, the niobium powder was rapid cooled to room temperature by moving it to cold zone. X-ray diffraction (XRD) analysis (Supplementary Fig. 2 ) indicated the obtained power consisted mainly of Nb, Nb 2 O 5 , and NbO. Ambient pressure CVD growth of NbSe 2 was conducted in a 2-inch outer diameter fused quartz tube heated by a Lindberg/Blue M (HTF55322C) split-hinge furnace. Supplementary Fig. 1 shows the set-up of the CVD reaction chamber. The partially oxidized Nb powders NbO x (0.7 g) together with NaCl powders (0.1 g) were placed in an alumina boat located in the center of the furnace. 285 nm SiO 2 /Si or other substrates were placed 1-3 mm above the powder mixture with the polished side faced down. Selenium powder (2 g) (99.5%, Sigma-Aldrich) was placed at the upstream of the quartz tube, where the temperature ranges from 300 to 460 °C during the reaction. 120 sccm (cubic centimeters per minute) Ar and 24 sccm H 2 are used as carrier gases. The furnace is heated to 795 °C in 16 min and maintained at that temperature for 13 min to allow the synthesis of NbSe 2 layers. The furnace was naturally cooled to 680 °C without changing the carrier gases. Then the top cover of the furnace was opened to allow fast cooling of the sample, with carrier gases switched to 250 sccm Ar and 4 sccm H 2 . Device fabrication and transport measurements For fabricating ultrathin NbSe 2 devices, large-area monolayer CVD graphene was used to cover and protect the thin NbSe 2 deposited on SiO 2 /Si. First, a rectangular frame consisted by adhesive tape was attached to the poly (methyl methacrylate) (PMMA)-coated graphene grown on Cu foil [50] . Then PMMA/graphene was detached from the Cu substrate by a bubbling transfer method. The PMMA/graphene was rinsed in DI water for several times and then dried in air. Second, the PMMA/graphene film was directly attached to the NbSe 2 on SiO 2 /Si substrate in an Ar-filled glove box, with the help of a drop of isopropanol added between. PMMA was then removed in acetone to form the graphene/NbSe 2 stacks. Finally, a fresh film of PMMA was deposited on the prepared graphene/NbSe 2 layers, by spin-coating at 3 K rpm for 1 min. The PMMA film was cured at 140 °C for 6 min in an Ar glove box. Hall bar device was made by electron-beam lithography and the contact metal (5 nm Cr/50 nm Au) was fabricated by electron-beam deposition. The transport experiment is carried out in a top-loading helium-3 cryostat in a superconducting magnet. An AC probe current I ac = 10 nA at 30.9 Hz is applied from the source to the drain. Then a lock-in amplifier monitors the longitudinal R xx through two additional electrical contacts. Fabrication of graphene/NbSe2/graphene sandwich cell for STEM imaging First, mono- and few-layer NbSe 2 crystals were grown on 285 nm SiO 2 /Si substrates. Second, with the same method described earlier in the device fabrication part, a continuous monolayer CVD graphene film was placed on top of the chip to form a graphene/NbSe 2 -stacked heterostructure. Third, a thin PMMA film was spin-coated and cured on the chip, and then the PMMA/graphene/NbSe 2 film was detached from the SiO 2 /Si substrate in HF. After rinsed in DI water, it was scooped up by a SiO 2 /Si chip predeposited with monolayer graphene film to form a PMMA/graphene/NbSe 2 /graphene structure on SiO 2 /Si substrate. Fourth, the PMMA/graphene/NbSe 2 /graphene film was detached from the substrate by etching SiO 2 layer in HF. After rinsed in DI water, it was scooped up by a TEM grid. Finally, the graphene/NbSe 2 /graphene sandwich cell was created by removing PMMA in acetone. Sample characterizations XPS spectra were collected on a PHI Quantera II spectrometer using monochromatic Al-Kα ( hυ = 1486.6 eV) radiation, and the binding energies were calibrated with C 1s binding energy of 284.8 eV. AFM images were taken using the Asylum Research Cypher AFM in tapping mode. Raman spectra were recorded in vacuum by a Witec system with ×50 objective lens and a 2400 lines per mm grating under 532 nm laser excitation. The laser power was fixed at 1 mW. STEM experiments were performed by a low acceleration voltage JEOL 2100F equipped with Delta correctors and GIF quantum spectrometer. Data availability The data that support the findings of this study are available from the corresponding author on reasonable request.